Crystalline-gradient polycarbonates prepared from enantioselective terpolymerization ofmeso-epoxides with CO2 The development of efficient processes for CO 2 transformation into useful products is a long-standing goal for chemists, since CO 2 is an abundant, inexpensive and non-toxic renewable C1 resource. Here we describe the enantioselective copolymerization of 3,4-epoxytetrahydrofuran with CO 2 mediated by biphenol-linked dinuclear cobalt complex, affording the corresponding polycarbonate with >99% carbonate linkages and excellent enantioselectivity (up to 99% enantiomeric excess). Notably, the resultant isotactic polycarbonate is a typical semicrystalline polymer, possessing a melting point of 271 °C. Furthermore, the enantioselective terpolymerization of 3,4-epoxytetrahydrofuran, cyclopentene oxide and CO 2 mediated by this dinuclear cobalt complex gives novel gradient polycarbonates, in which the decrement of one component and the increment of the other component occur sequentially from one chain end to the other end. The resultant terpolymers show perfectly isotactic structure and have unique crystalline-gradient nature, in which the crystallinity continuously varies along the main chain. The utilization of carbon dioxide (CO 2 ) as a C1 source for the production of useful chemicals has received intense attention in recent decades [1] , [2] , [3] , [4] , [5] . This is motivated by the economic and environmental benefits arising from the use of the abundant renewable resource and the growing concern on the greenhouse effect. Conforming to this objective, the alternating copolymerization of CO 2 with epoxides for the synthesis of degradable polycarbonates is one of the most promising green reactions, which was first demonstrated by Inoue et al. [6] Subsequent to the early discovery, numerous heterogeneous and well-defined homogeneous catalysts have been developed for this important transformation [7] , [8] , [9] , [10] , [11] , [12] , [13] . Despite the tremendous progress made in this field, most of the CO 2 -based polycarbonates are known to be amorphous, and their low thermal resistance makes them difficult to use as structural materials. In a recent study, we reported a typical semicrystalline polymer, isotactic poly(cyclohexene carbonate), prepared by enantioselective copolymerization of CO 2 with meso cyclohexene oxide [14] . It was also found that the isotacticity had the critical influence on the crystallinity of poly(cyclohexene carbonate)s. Following this investigation, several crystalline CO 2 -based polycarbonates with good thermal stability were discovered [15] , [16] , [17] . Since the relative stereochemistry of adjacent stereocentres in a defined polymer has a significant effect on its thermal and physical properties, precise control of a polymer’s stereoregularity is an important goal in polymerization catalysis [18] . Recently, Kamigaito’s group [19] , [20] reported a new class of polymers, stereogradient polymers, produced from the stereospecific living radical copolymerization of two monomers with different reactivities and stereospecificities. In these stereogradient polymers, the tacticity continuously changes from one chain end to the other end, unlike traditional stereo-block or -random copolymers. Following their excellent catalyst design of salen-type cobalt complex with a piperidinium end-capping arm [21] , Nozaki and coworkers [22] reported a novel stereogradient, poly(propylene carbonate)s (PPCs), consisting of two enantiomeric structures on each end, prepared by this cobalt complex-mediated regio- and enantioselective copolymerization of racemic propylene oxide with CO 2 . The iso-enriched stereogradient PPC starts from an ( S )-rich PPC block and ends with an ( R )-rich PPC block. Notably, the obtained stereogradient PPCs were found to possess higher thermal decomposition temperature than the typical PPCs [23] . Herein, we describe a synthetic strategy of preparing crystalline-gradient polycarbonates by dinuclear cobalt(III) complex-mediated enantioselective terpolymerization of meso -3,4-epoxytetrahydrofuran (COPO), cyclopentene oxide (CPO) and CO 2 , in which two epoxides have different reactivities in terpolymerizing with CO 2 . Crystalline-gradient polycarbonates can be defined as polymers in which the crystallinity sequentially varies along the main chain and have never been reported previously. Synthesis of isotactic polycarbonates from COPO Meso -COPO, consisting of a three-membered epoxy-ring and a five-membered ring with one oxygen atom, perhaps has a relatively high reactivity in coupling with CO 2 by its epoxy-ring in the presence of a metal catalyst, while the oxygen atom in the five-membered ring makes it have obvious difference in comparison with CPO, a previously studied meso -epoxide [24] . Recently, we developed a chiral catalyst system based on the biphenol-linked dinuclear Co(III) complex ( Fig. 1 ), which exhibited excellent activity, unprecedented enantioselectivity and molecular-weight control for the alternating copolymerization of CO 2 with meso -epoxides such as CPO under mild reaction conditions [25] . Previously, Coates and co-workers [26] , [27] , [28] have demonstrated that the dinuclear cobalt complexes based on binaphthol linker were highly active and enantioselective for homopolymerization of terminal epoxides. As a consequence, the same enantiopure biphenol-linked dinuclear Co(III) complex was employed as catalyst for enantioselective copolymerization of CO 2 with COPO. As expected, the catalyst exhibited excellent enantioselectivities under mild conditions. 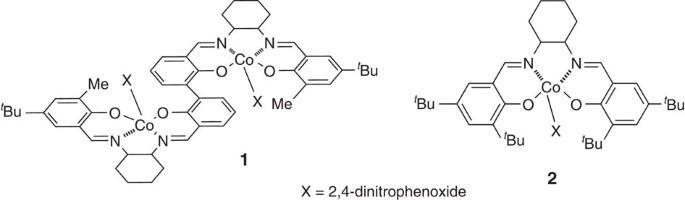Figure 1: Structure of Co(III)–Salen complex. Full synthesis procedure and characterization are provided in theSupplementary Methods. The screening experimental results are summarized in Table 1 . The dinuclear cobalt complex ( S,S,S,S )- 1 alone as catalyst could catalyse the coupling reaction at room temperature to afford the corresponding copolymer with 85% enantioselectivity for S,S -configuration excess, although the activity was not satisfactory ( Table 1 , entry 1). The copolymer enantioselectivity is based on the enantiomeric excess (ee) of the dibenzoate of the diol that resulted from the hydrolysis of the resultant polycarbonates, as determined by chiral high-performance liquid chromatography ( Supplementary Methods ). The presence of PPNX (PPN=bis(triphenylphosphine)iminium, X=2,4-dinitrophenoxide) as cocatalyst significantly improved both activity (a turnover frequency (TOF) of 170 h −1 ) and enantioselectivity (95% ee) (Entry 2). It should be noted that the resultant copolymers possess perfectly alternating nature with >99% carbonate unit content ( Fig. 2 and Supplementary Fig. 1 ) and neither the cyclic carbonate byproduct nor the polyether linkage was found in the two systems. The reaction temperature has a strong influence on both enantioselectivity and activity for this asymmetric copolymerization process. For example, when the reaction temperature decreased from 25 to 0 °C, the enantioselectivity of the resulting polycarbonates increased from 95% to 99% ( Table 1 , entry 3 and Supplementary Figs 6 and 7 ). Similar activity and enantioselectivity were also observed in the ( R,R,R,R )- 1 -mediated CO 2 /COPO copolymerization, providing the copolymer with R,R -configuration absolutely (Entry 4). When the dinuclear cobalt catalyst system was performed at 50 °C, providing a completely alternating copolymer with an enantioselectivity of 90% ee for S , S -configuration, the activity was increased to 458 h −1 (Entry 5). On increasing the [COPO]/[( S,S,S,S )- 1 ] ratio from 1,000 to 2,000, the TOF was decreased from 170 to 132 h −1 ; however, the enantioselectivity was maintained at a high level (Entry 6). Especially, with the use of dichloromethane as an organic solvent, the complete conversion of epoxide was achieved in a prolonged time at room temperature, affording the polycarbonates with an enantioselectivity of 98% ee for S , S -configuration ( Table 1 , entry 7 and Supplementary Fig. 2 ). Figure 1: Structure of Co(III)–Salen complex. Full synthesis procedure and characterization are provided in the Supplementary Methods . Full size image Table 1 Enantiopure Co(III)-complex-mediated asymmetric copolymerization CO 2 with COPO * . 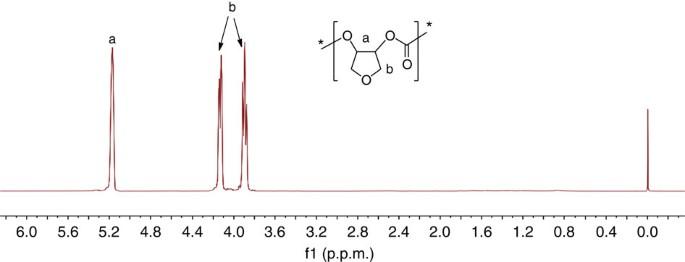Figure 2:1H NMR spectrum ofa representative sample of PCOPC in CDCl3. The polymer was purified by using DMSO/MeOH. (a) Methine hydrogen atoms; (b) methylene hydrogen atoms. * Repeat carbonate unit of polymers. Full size table Figure 2: 1 H NMR spectrum of a representative sample of PCOPC in CDCl 3 . The polymer was purified by using DMSO/MeOH. (a) Methine hydrogen atoms; (b) methylene hydrogen atoms. * Repeat carbonate unit of polymers. Full size image For comparison, the atactic CO 2 /COPO copolymer (PCOPC) was prepared using an irregular rac - 2 /PPNX (X=2,4-dinitrophenoxide) catalyst system ( Table 1 , entry 8 and Supplementary Fig. 3 ). Although the accurate assignation of the microstructure of this polycarbonate proved to be very difficult, 13 C NMR study could clearly reveal the significant difference in the methine region between the atactic and highly isotactic copolymers ( Supplementary Fig. 4 ). Being different from the previous poly(cyclohexene carbonate)s and poly(cyclopentene carbonate)s (PCPC), the carbonyl group of the PCOPC showed negligible differences between the atactic and isotactic copolymers. The crystallization and melting behaviour of the polycarbonates were studied by means of differential scanning calorimetry (DSC) in a flowing nitrogen atmosphere. Only a single glass transition peak was observed at around 122 °C for the atactic copolymers ( Fig. 3 , left plot, curve A). As the isotacticity of PCOPC has a critical influence on its crystallinity, it was found that the polycarbonates with moderate isotacticity (ee=85%) gave a weak T g of 125 °C and a melting endothermic peak at 265 °C with the melting enthalpy (Δ H m ) of 25.21 J g −1 ( Fig. 3 , left plot, curve C). Regarding the highly isotactic copolymer with >99% ee, one should first notice that the T g peak has disappeared completely, while a quite sharp and high crystallization endothermic peak is found at 271 °C with Δ H m =32.24 J g −1 ( Fig. 3 , left plot, curve B), indicating a very high degree of crystallinity. Furthermore, the crystallization behaviour of highly isotactic polycarbonates was also confirmed by the wide-angle X-ray diffraction (WAXD) study. No diffraction was observed for the corresponding atactic copolymer, confirming its amorphous feature ( Fig. 3 , right plot, curve A). On the contrary, for highly isotactic ( S )-copolymers, sharp diffraction peaks were observed at 2 θ values of 18.1°, 19.9° and 23.2°, demonstrating that the isotactic copolymer was a typical semicrystalline polymer ( Fig. 3 , right plot, curve B). As expected, the thermo-gravimetric analysis revealed that the resulting polymer exhibited excellent thermal stability with a thermolysis temperature >300 °C ( Supplementary Fig. 5 and Supplementary Methods ). 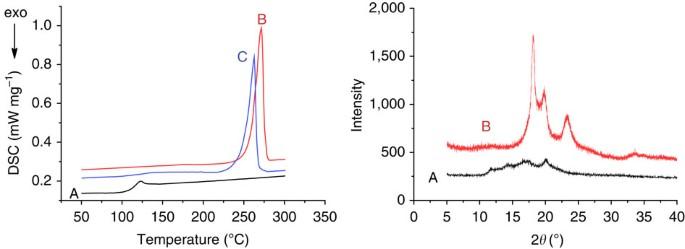Figure 3: DSC thermograms and WAXD profiles of various PCOPCs. DSC thermograms (left) in second heating and WAXD profiles (right) of (A) atactic PCOPC (ee=0%,Table 1, entry 8), (B) highly isotactic PCOPC (ee>99%,Table 1, entry 3) and (C) PCOPC with moderate isotacticity (ee=85%,Table 1, entry 1). The PCOPCs undergo end-capping reaction. Experimental procedures for end-capping reaction and conditions of DSC and WAXD analysis are all described inSupplementary Methods. Figure 3: DSC thermograms and WAXD profiles of various PCOPCs. DSC thermograms (left) in second heating and WAXD profiles (right) of (A) atactic PCOPC (ee=0%, Table 1 , entry 8), (B) highly isotactic PCOPC (ee>99%, Table 1 , entry 3) and (C) PCOPC with moderate isotacticity (ee=85%, Table 1 , entry 1). The PCOPCs undergo end-capping reaction. Experimental procedures for end-capping reaction and conditions of DSC and WAXD analysis are all described in Supplementary Methods . Full size image Synthesis of crystalline-gradient polycarbonates Although the terpolymerization of CO 2 with alicyclic or/and aliphatic epoxides was frequently reported using various organometallic catalysts [29] , [30] , [31] , [32] , [33] , the synthesis of high stereoregular or crystallizable CO 2 -based terpolymers was never reported as a consequence of the lack of a highly enantioselective catalyst [34] . Since enantiopure dinuclear cobalt complex 1 is an excellent privileged catalyst for enantioselective copolymerization of CO 2 with various meso -epoxides, it was applied to the terpolymerization of CO 2 , COPO and CPO. As expected, the binary ( S,S,S,S )- 1 /PPNX (X=2,4-dinitrophenoxide) catalyst system showed high activity for CO 2 /COPO/CPO terpolymerization at various epoxide ratios in the feedstock under 25 °C, selectively providing the terpolymers with different composition ( Table 2 ). In the 1 H NMR spectrum of the resulting terpolymers in deuterated chloroform, the resonance of methine CH in the COPC unit is located at 5.30 p.p.m., whereas the CH in the cyclopentene carbonate (CPC) unit is located at 5.02 p.p.m. ( Supplementary Figs 8–10 ). Moreover, neither the polyether structure nor cyclic carbonate was detected during the terpolymerization. Notably, the enantioselectivity for COPC and CPC units in the terpolymers was the same as that found in the polycarbonates that resulted from the copolymerization of COPO or CPO alone with CO 2 . For example, the ee of cyclopentane-1,2-diol and tetrahydrofuran-3,4-diol that resulted from the CO 2 /COPO/CPO terpolymer was 99% and 95% for ( S,S )-configuration, respectively, which is in accordance with the copolymerization described in Table 2 , entries 1 and 2. Table 2 CO 2 /COPO/CPO terpolymerization mediated by ( S,S,S,S )-1/PPNX catalyst system * . Full size table Surprisingly, COPO and CPO exhibited comparable reactivities in copolymerizing with CO 2 catalysed by ( S,S,S,S )- 1 /PPNX (X=2,4-dinitrophenoxide) system, but a marked difference in reactivity was observed in the CO 2 /COPO/CPO terpolymerization ( Table 2 ). From the competition polymerization of COPO and CPO with CO 2 using various epoxide feed ratios at room temperature, monomer reactivity ratios could be obtained ( r COPO =8.49 and r CPO =0.17) ( Fig. 4 and Supplementary Table 1 ). These data indicated a much higher activity for the synthesis of COPC–COPC linkages at the initial stage owing to the lower reactivity of CPO in the terpolymerization. The terpolymers with various COPC unit contents showed different melting behaviours, and the T m was associated with the proportion of COPC unit content in the polymer ( Fig. 5 ). When the COPC unit content was 98%, the terpolymer showed a T m of 265 °C ( Fig. 5 , curve E). With decrease in the COPC unit content in the terpolymers, T m was also decreased gradually and the appearance of a T g was more and more obvious. When the COPC unit content was decreased to 30.6%, the terpolymer became an amorphous material with a T g of 89 °C ( Fig. 5 , curve A), close to the T g of the isotactic PCPC. It should be noted that a T m of 270 °C and a T g of 84 °C were detected in the blend of equivalent, isotactic ( S )-PCPC and ( S )-PCOPC ( Fig. 5 , curve F). 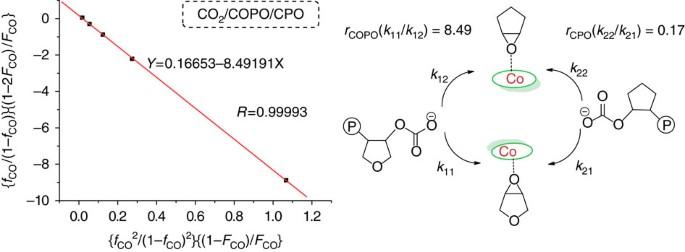Figure 4: Fineman–Ross plot and kinetic parameters for terpolymerization of COPO/CPO/CO2by the dinuclear cobalt/PPNX catalyst system. Experimental data are described inSupplementary Table 1. Figure 4: Fineman–Ross plot and kinetic parameters for terpolymerization of COPO/CPO/CO 2 by the dinuclear cobalt/PPNX catalyst system. Experimental data are described in Supplementary Table 1 . 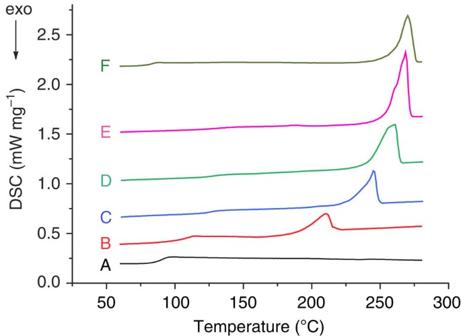Figure 5: DSC profiles of CO2/COPO/CPO terpolymers. (A) With 30.6% COPC unit content (Table 2, entry 3), (B) with 69.0% COPC unit content (entry 4), (C) with 84.2% COPC unit content (entry 5), (D) with 92.3% COPC unit content (entry 6), (E) with 98.0% COPC unit content (entry 7), (F) blend of (S)-PCPC (ee>99%,Table 2, entry 2)/(S)-PCOPC (ee>99%,Table 1, entry 3), 1/1 mass ratio. Full size image Figure 5: DSC profiles of CO 2 /COPO/CPO terpolymers. (A) With 30.6% COPC unit content ( Table 2 , entry 3), (B) with 69.0% COPC unit content (entry 4), (C) with 84.2% COPC unit content (entry 5), (D) with 92.3% COPC unit content (entry 6), (E) with 98.0% COPC unit content (entry 7), (F) blend of ( S )-PCPC (ee>99%, Table 2 , entry 2)/( S )-PCOPC (ee>99%, Table 1 , entry 3), 1/1 mass ratio. Full size image In order to determine the relationship between the COPC unit content in the terpolymers and the reaction time, 1 H NMR analysis was used to track the polymerization process by the intermittent sampling experiments. The terpolymerization was carried out with equimolar COPO and CPO in dichloromethane solution at 25 °C. COPO was predominantly copolymerized with CO 2 at the beginning stage of the reaction because of its relative high reactivity, while CPO was incorporated into the terpolymer mainly at the high conversions ( Fig. 6 , plot-(a)). Since ( S,S,S,S )- 1 /PPNX-mediated CO 2 / meso -epoxide copolymerization or terpolymerization exhibits a living polymerization character, a gradient distribution of COPC and CPC units in the terpolymers was formed. The decrement of COPC carbonate unit and the increment of CPC unit occur sequentially from one chain end to the other end, unlike traditional block or random copolymers ( Fig. 7 ). As previously mentioned, highly isotactic PCOPCs are typical semicrystalline polymers, while both isotactic and atactic PCPCs are amorphous. As a result, the COPO/CPO/CO 2 terpolymers with gradient distribution might show a unique crystalline-gradient nature. This means that the crystallinity varies continuously along the main chain, and the thermal properties of the terpolymers should depend on the COPC carbonate unit content. For example, when the reaction was performed for 8 h, the terpolymers with the 83% COPC carbonate unit showed a T m of 245 °C ( Fig. 6 , plot-(b), curve A). With the increment of the reaction time, the Δ H m ascribed to PCOPC was reduced and the T g ascribed to PCPC and/or incorporated with minor COPC units appeared. After 36 h, the complete conversion of all epoxides was achieved, and the resultant terpolymers had a T m of 241 °C and a T g of 106 °C ( Fig. 6 , plot-(b), curve C). Especially, the isolated terpolymers that resulted from various time points all have narrow molecular weight distributions (<1.2) and exhibit perfectly monomodal distribution. Although the M n ’s are lower than the expected values, a linear relationship between the conversion of epoxide and M n of the resultant copolymers was found, which was consistent with the immortal polymerization characteristic ( Fig. 6 , plots-(c) and (d)) [35] . However, it is worth noting here that the adventurous water or the addition of a protic agent such as methanol can cause chain transfer, thus resulting in the reduced molecular weight. 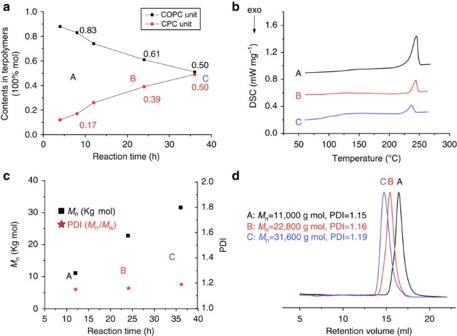Figure 6: Analysis of gradient polycarbonates. (a) Plot of the COPC and CPC carbonate unit contents in the resulting terpolymers versus the reaction time in the COPO/CPO/CO2terpolymerization catalysed by (S,S,S,S)-1/PPNX system in dichloromethane (epoxide/dichloromethane=1/2 (molar ratio),1/PPNX/COPO/CPO=1/2/250/250 (molar ratio), X=2,4-dinitrophenoxide) at 25 °C. (b) DSC profiles of gradient terpolymers at various time points: (A) 8 h; (B) 24 h; (C) 36 h. (c) Plots of the terpolymer molecular weight and distribution versus the reaction time. (d) GPC traces of the COPO/CPO/CO2terpolymers obtained at various time points: (A) 8 h; (B) 24 h; (C) 36 h. Figure 6: Analysis of gradient polycarbonates. ( a ) Plot of the COPC and CPC carbonate unit contents in the resulting terpolymers versus the reaction time in the COPO/CPO/CO 2 terpolymerization catalysed by ( S,S,S,S )- 1 /PPNX system in dichloromethane (epoxide/dichloromethane=1/2 (molar ratio), 1 /PPNX/COPO/CPO=1/2/250/250 (molar ratio), X=2,4-dinitrophenoxide) at 25 °C. ( b ) DSC profiles of gradient terpolymers at various time points: (A) 8 h; (B) 24 h; (C) 36 h. ( c ) Plots of the terpolymer molecular weight and distribution versus the reaction time. 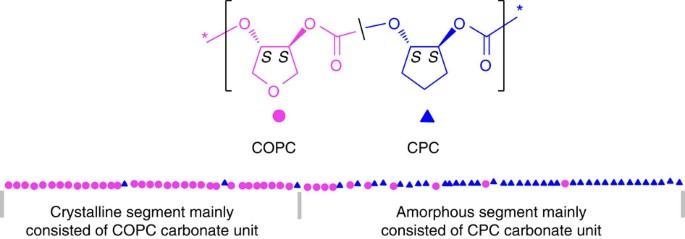Figure 7: Crystalline-gradient polycarbonates that resulted from CPO/COPO/CO2terpolymerization. Decrement of COPC carbonate unit and increment of CPC unit occur sequentially from one chain end to the other end. * Repeat carbonate unit of polymers. ( d ) GPC traces of the COPO/CPO/CO 2 terpolymers obtained at various time points: (A) 8 h; (B) 24 h; (C) 36 h. Full size image Figure 7: Crystalline-gradient polycarbonates that resulted from CPO/COPO/CO 2 terpolymerization. Decrement of COPC carbonate unit and increment of CPC unit occur sequentially from one chain end to the other end. * Repeat carbonate unit of polymers. Full size image In conclusion, we have demonstrated that the highly isotactic polycarbonate produced from the dinuclear cobalt complex-mediated enantioselective copolymerization of CO 2 with 3,4-epoxytetrahydrofuran is a typical semicrystalline thermoplastic, and possesses a high T m of 271 °C with Δ H m =32.24 J g −1 . Also, the catalyst system was proved to be very effective in the enantioselective terpolymerization of COPO, CPO and CO 2 , affording the terpolymers with gradient distribution of two kinds of carbonate units. The resultant terpolymers have unique crystalline-gradient nature, in which the crystallinity varies continuously along the main chain. Further study will focus on the terpolymerization of other meso -epoxides and develop more versatile CO 2 -based polycarbonates with morphology structure. General All manipulations involving air- and/or water-sensitive compounds were carried out in a glove box or with the standard Schlenk techniques under dry nitrogen. CO 2 (99.995%) was purchased from the Dalian Institute of Special Gases and used as received. Methylene chloride and DMSO were distilled from calcium hydride under nitrogen. CPO and COPO were purchased from Acros and distilled over calcium hydride. Procedures for copolymerizing CO 2 with COPO In a predried 20 ml autoclave equipped with a magnetic stirrer, dinuclear cobalt catalyst (0.030 mmol, 1 equiv) and PPNX (0.060 mmol, 2 equiv, X=2,4-dinitrophenoxide) were dissolved in COPO (30 mmol, 1,000 equiv) in an argon atmosphere. CO 2 was introduced into the autoclave for a designed pressure. The reaction mixture was stirred at a desired temperature for an appropriate time. After the allotted reaction time, CO 2 was released, and the unreacted COPO was isolated under reduced pressure. A small amount of the resultant mixture was removed for 1 H NMR analysis to quantitatively give the selectivity of polycarbonate to cyclic carbonate, as well as carbonate linkages. The crude polymer was dissolved in 10 ml DMSO and precipitated from methanol. This process was repeated 3–5 times to completely remove the catalyst, and white polymer was obtained by vacuum-drying. Synthetic procedure of gradient terpolymer In a predried 20 ml autoclave equipped with a magnetic stirrer, dinuclear cobalt catalyst 1 (0.030 mmol, 1 equiv) and PPNX (0.060 mmol, 2 equiv, X=2,4-dinitrophenoxide) were dissolved in COPO and CPO (1/1 molar ratio, 15 mmol, 500 equiv), and CH 2 Cl 2 (2 ml) was added to the mixture under an argon atmosphere. CO 2 was introduced into the autoclave for a designed pressure. The reaction mixture was stirred at a desired temperature for the appropriate time. Then CO 2 was released, and a small amount of the resultant mixture was removed from the autoclave for 1 H NMR analysis to quantitatively give the selectivity of the polymer to cyclic carbonates, and carbonate linkages, as well as the composition of COPC and CPC units in the resultant terpolymers. The crude terpolymer was dissolved in 10 ml DMSO and precipitated from methanol. This process was repeated 3–5 times to remove the catalyst, and white terpolymer was obtained by vacuum-drying. The resultant terpolymer was used for GPC and DSC analysis. How to cite this article: Liu, Y. et al. Crystalline-gradient polycarbonates prepared from enantioselective terpolymerization of meso -epoxides with CO 2 . Nat. Commun. 5:5687 doi: 10.1038/ncomms6687 (2014).